High-resolution structure of theShigellatype-III secretion needle by solid-state NMR and cryo-electron microscopy We introduce a general hybrid approach for determining the structures of supramolecular assemblies. Cryo-electron microscopy (cryo-EM) data define the overall envelope of the assembly and rigid-body orientation of the subunits while solid-state nuclear magnetic resonance (ssNMR) chemical shifts and distance constraints define the local secondary structure, protein fold and inter-subunit interactions. Finally, Rosetta structure calculations provide a general framework to integrate the different sources of structural information. Combining a 7.7-Å cryo-EM density map and 996 ssNMR distance constraints, the structure of the type-III secretion system needle of Shigella flexneri is determined to a precision of 0.4 Å. The calculated structures are cross-validated using an independent data set of 691 ssNMR constraints and scanning transmission electron microscopy measurements. The hybrid model resolves the conformation of the non-conserved N terminus, which occupies a protrusion in the cryo-EM density, and reveals conserved pore residues forming a continuous pattern of electrostatic interactions, thereby suggesting a mechanism for effector protein translocation. Large molecular assemblies are omnipresent in living cells and responsible for a broad spectrum of biological functions, such as cellular motion (molecular motors), cellular structure (cytoskeletal filaments) and molecular transport (bacterial secretion systems). Traditionally, X-ray crystallography, solution-state nuclear magnetic resonance (NMR) and cryo-electron microscopy (cryo-EM) are used to probe the atomic structures of biomolecular systems. Molecular assemblies, however, pose technical challenges for conventional methods [1] : finding an appropriate crystallization condition is a strenuous effort for large, multi-subunit systems; crystallization can be prevented by the presence of flexible or disordered regions or domains; and systems with non-crystallographic symmetry lack the long-range order required to produce a discrete diffraction pattern. In addition, high-molecular weight (MW) protein complexes (in excess of 100 kDa) generally do not exhibit sufficiently fast molecular tumbling to be studied by solution-state NMR spectroscopy, with notable exceptions for favourable systems [2] . The study of isolated structural domains at atomic resolution is insufficient for a complete description of the larger, biologically active system, as proteins can adopt different conformations in isolation compared with their functional complexes. Two methods are emerging to tackle the structures of intact large assemblies towards gaining a mechanistic insight into their biological function. Technically, both solid-state NMR [3] , [4] , [5] , [6] (ssNMR) and cryo-EM [7] , [8] are not limited by the molecular size of the assembly under study. Density data from cryo-EM defines an overall envelope of the supramolecular assembly in a resolution range of 20–8 Å for standard applications and up to 4 Å for favourable systems [1] . ssNMR data provide crucial information on the local structure such as the secondary structure propensity, backbone dihedral angles and inter-atomic distances of up to ~10 Å, which can be detected both within the individual protein domains and across inter-molecular subunit interfaces. Cryo-EM and ssNMR data are in principle highly complementary and their use in combination holds great promise for future hybrid structural studies [9] . However, a general framework to integrate the different sources of structural information into high-resolution models of multimeric assemblies has been limited by (1) the different levels of resolution provided by each technique that complicates their use in computational methods, the fine-tuning of relative constraint weights and the assessment of self-consistency between these fundamentally different data sets and (2) the availability of computational methods that would determine the range of models consistent with the experimental data, as a function of the varying degrees of freedom. We introduce a generalized hybrid approach for high-resolution structure determination of supramolecular assemblies that combines high-resolution cryo-EM density maps with ssNMR distance constraints. We demonstrate the power of the new approach by determining the structure of the type-III secretion system (T3SS) needle of Shigella flexneri at atomic resolution (to a precision of 0.4 Å backbone r.m.s.d.). The T3SS, or injectisome, is a supramolecular assembly found in Gram-negative bacteria, such as Shigella , Salmonella , Escherichia , Pseudomonas or Yersinia [10] , which serves to deliver toxic effector proteins into their target eukaryotic host cell during infection [11] , [12] . The current study extends and improves on our previous work focusing on T3SS needles, which include the atomic model of Salmonella typhimurium [13] , [14] , [15] using ssNMR data and helical parameters from scanning transmission electron microscopy (STEM), the ssNMR resonance assignment of Shigella flexneri MxiH needles [16] , which allowed to identify a common architecture for T3SS needles, the study of dynamics and conformational heterogeneity of MxiH needles using dynamic nuclear polarization-enhanced ssNMR [17] , and ssNMR assignment strategies using sparsely 13 C-labelled samples [18] , [19] , [20] or highly deuterated proteins [21] . The new hybrid approach combines a 7.7-Å cryo-EM density map reconstructed using 100,000 needle segment images [22] with extensive structural information obtained from ssNMR: 162 backbone dihedral angles and 996 carbon–carbon distance constraints from proton-driven spin diffusion (PDSD [23] , [24] ) experiments. The calculated structures are validated using 691 independent distance constraints: carbon–carbon constraints from PDSD experiments and proton–proton constraints from ChhC and NhhC experiments ( 13 C– 13 C and 15 N– 13 C proton-mediated correlation spectrum, respectively) [25] , [26] . With 12 and 8 distance constraints per residue in the calculation and validation sets, respectively, the final models are among the most well-resolved ssNMR structures to date [27] , [28] . Moreover, the atomic structures reveal the conformation of the previously undefined N-terminal segment (residues 1–11) and provide new insight into the protein translocation mechanism. Identification of the fold and inter-molecular interfaces We have previously achieved the NMR chemical-shift assignment of MxiH needles [16] , which allowed us to identify the secondary structure of MxiH subunit proteins in their assembled state. In that work, we employed ssNMR experiments having short mixing times (for example, PDSD ≤100 ms) to obtain intra-residue and sequential amino-acid connectivity information. 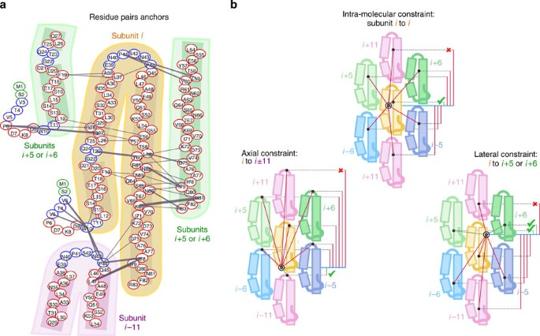Figure 1: Preliminary map of theShigella flexnerineedle architecture. (a) Anchor point identification in the absence of previous structural knowledge. Proximity anchors are identified by at least two unambiguous (corresponding to well-resolved and readily assigned cross-peaks) or abundant (≥4) contacts in spectra of [1-13C]-glucose- and [2-13C]-glucose-labelled MxiH needles (gray lines, line thickness proportional to the number of contacts). (b) Strategy for assignment of ssNMR constraints arising from distinct intra-molecular and inter-molecular interfaces in helical assemblies. Pink lines indicate interface assignments of a given contact that are inconsistent with the axial displacement among symmetry-related subunits, and green lines the correct interface assignments. In the current work, we recorded a set of diverse and complementary experiments employing long PDSD mixing times (400–850 ms) that provided a large number of cross-peaks corresponding to medium and long-range distance constraints ( Supplementary Table 1 ). Experiments were recorded on [1- 13 C]-glucose (1-Glc)- and [2- 13 C]-glucose (2-Glc)-labelled protein samples. Additional ChhC and NhhC experiments [25] , [26] were recorded on a uniform 13 C-labelled sample. To favour the detection of long-range cross-peaks, we recorded individual spectra with high signal-to-noise ratio. From the 1-Glc and 2-Glc sets of spectra, we can rapidly identify pairs of amino acids called anchor points, which are certain to be in close distance proximity using two telltale spectral features: (1) frequency-unambiguous cross-peaks have only one possible NMR assignment within a ±0.15-p.p.m. tolerance window; (2) network-unambiguous cross-peaks are part of an extensive network with numerous distance constraints between two amino acids. These anchor points, combined with the previously established secondary structure [16] , serve to define the main fold of the MxiH subunits in the context of the needle assembly de novo , without using any previous structural model. In detail, amino-acid pairs related by at least two frequency-unambiguous cross-peaks or by four or more cross-peaks in a given labelling scheme are used as anchors to produce a preliminary map of the Shigella needle architecture ( Fig. 1a ). A cluster of contacts between the two antiparallel α-helices (for example, F19-A63/Q64, T23-Y60 and L26/Q27-Y57) indicates that MxiH subunits adopt a typical helix-loop-helix fold. Residues N43, P44 and L47 in the loop region make contacts with the end of the C-terminal α-helix (for example, P44-I78, L47-I78/79) as well as with the rigid N-terminal segment (W10-N43/P44), indicating that subunit ( i ) and subunit ( i −11) of the helical assembly are arranged in a head-to-tail manner, forming an inter-molecular axial interface. An extensive lateral interface comprises a dense network of contacts formed between the C-terminal regions L59-K69 of subunit ( i ) and K72-R83 of subunits ( i +5) and ( i +6). Lateral contacts are also found between the loop region and both the N-terminal helix (F19-L37/A38) and the C-terminal helix (P41-L59/Y60). The rigid N-terminal extension (S2 to T11) is curved, as indicated by multiple contacts between tryptophan W10 and N-terminal residues V3–V5. Further contacts (P6-Q27/G28) indicate a lateral inter-molecular association between the N-terminal extension and the central region of the N-terminal helix that forms a minor kink at residues G22–Q24. This map confirms that the protein fold and inter-molecular interfaces identified in Salmonella typhimurium T3SS needles [13] are also present in Shigella flexneri needles. Figure 1: Preliminary map of the Shigella flexneri needle architecture. ( a ) Anchor point identification in the absence of previous structural knowledge. Proximity anchors are identified by at least two unambiguous (corresponding to well-resolved and readily assigned cross-peaks) or abundant (≥4) contacts in spectra of [1- 13 C]-glucose- and [2- 13 C]-glucose-labelled MxiH needles (gray lines, line thickness proportional to the number of contacts). ( b ) Strategy for assignment of ssNMR constraints arising from distinct intra-molecular and inter-molecular interfaces in helical assemblies. Pink lines indicate interface assignments of a given contact that are inconsistent with the axial displacement among symmetry-related subunits, and green lines the correct interface assignments. Full size image Assignment of a large number of distance constraints Using the preliminary map, we proceed to the disambiguation of all ssNMR distance constraint cross-peaks collected in the 1-Glc and 2-Glc spectra. The use of sparse 13 C-labelling schemes enables very high spectral resolution, with 13 C line-widths ranging from 0.09 to 0.25 p.p.m., and the high spectral homogeneity of the T3SS needle samples leads to very small assignment uncertainty, with the s.d. of intra-residue and sequential peak positions over all spectra of 0.04 p.p.m. on average for 13 C and 0.03 p.p.m. for 15 N. To further improve the accuracy of the chemical-shift assignment for long mixing-time experiments, we re-calculated the full table of average resonance frequencies on an individual basis for each dimension of each spectrum, when enough intra-residue and sequential cross-peaks were available. A Sparky extension was created to display per spectrum resonance frequencies and a robust estimate of the average frequency ( Supplementary Software 1 ). Our method thus allows the use of small tolerance windows (±0.15 p.p.m. for 13 C chemical shifts), which results in a drastic reduction of the number of assignment possibilities for each cross-peak. Assignment ambiguity exists at two levels, chemical-shift ambiguity and subunit ambiguity. Chemical-shift ambiguity relates to the identification of carbon nuclei that give rise to the cross-peak. Subunit ambiguity exists as each cross-peak can arise due to either of one intra-subunit and six different inter-subunit atom-pair combinations ( Fig. 1b ): intra-subunit, ( i ) to ( i ); inter-subunit, lateral: ( i ) to ( i ±5) or ( i ) to ( i ±6); and inter-subunit, axial: ( i ) to ( i ±11). The presence of multiple, distinct interfaces could potentially complicate the subunit-subunit assignment of ssNMR constraints. However, it is possible to exploit the particular architecture of helical assemblies, as the symmetry of the structure dictates that subunits ( i ±5) and ( i ±6) are located within one axial translation (L) relative to subunit ( i ), and subunits ( i ±11) within two axial translations ( Fig. 1b ). This approach eliminates the need to produce an additional mixed isotopically labelled sample for the purpose of interface identification [29] , [30] . In the more general case, helical assemblies consist of layers of subunits with axial translations of 0, 1 and 2: for example, for an alternative 13-start helical assembly, subunits ( i ), ( i ±6/7) and ( i ±13) have axial translations of 0, ±1 and ±2, respectively. Our approach can thus be applied to any helical arrangement of subunits regardless of the number of subunits per layer. As demonstrated in Fig. 1b , we can utilize the short axial translation between two amino-acid pairs in the preliminary map to classify a distance constraint as intra-molecular, axial or lateral in the absence of a preliminary structural model of the system. Chemical-shift ambiguities that do not fit any of the three inter-subunit categories are also excluded, allowing further disambiguation of cross-peaks. One type of subunit ambiguity remains, however, for lateral constraints, as subunits ( i ±5) and ( i ±6) have similar axial translations within the assembly, and is resolved in the iterative approach presented below. The distance constraints collected from the 1-Glc and 2-Glc spectra were classified as unambiguous if the chemical-shift ambiguities could be adequately resolved (total of 1,190 correlations), or as ambiguous cross-peaks otherwise ( Fig. 2 ). Ambiguous correlations and correlations from the uniformly 13 C/ 15 N-labelled data set (ChhC and NhhC) were reserved to be used for cross-validation of the final models (as outlined in the structure validation section). 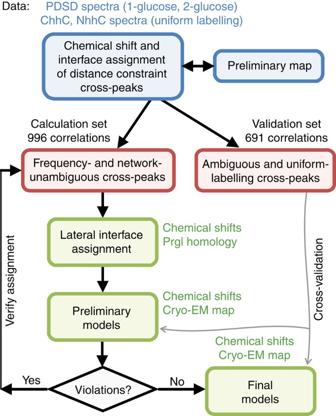Figure 2: Flowchart of the iterative assignment/structure determination process. Flowchart presenting the assignment procedure of ssNMR distance constraints and structural modelling in the new hybrid approach. Steps of NMR data analysis are coloured blue, with the resulting data sets illustrated as red rectangles. Rosetta-modelling steps are coloured green and the additional data used at each modelling step are indicated, including the 7.7-Å cryo-EM density map22. The preliminary models are derived from a reduced set of distance constraints coming only from [2-13C]-glucose spectra. The final models employ distance constraints from all data sets. The use of the software tools performing the different steps in the flow chart (provided asSupplementary Software 1) is outlined in detail inSupplementary Methods. Figure 2: Flowchart of the iterative assignment/structure determination process. Flowchart presenting the assignment procedure of ssNMR distance constraints and structural modelling in the new hybrid approach. Steps of NMR data analysis are coloured blue, with the resulting data sets illustrated as red rectangles. Rosetta-modelling steps are coloured green and the additional data used at each modelling step are indicated, including the 7.7-Å cryo-EM density map [22] . The preliminary models are derived from a reduced set of distance constraints coming only from [2- 13 C]-glucose spectra. The final models employ distance constraints from all data sets. The use of the software tools performing the different steps in the flow chart (provided as Supplementary Software 1 ) is outlined in detail in Supplementary Methods . Full size image Owing to the high spectral resolution and signal-to-noise ratio of the ssNMR data, a large number of distance constraints can be found for individual nuclei. More than 12,350 cross-peaks were analysed in long-range spectra and over 17,850 cross-peaks were analysed in total, including short mixing-time spectra. Excerpts from PDSD spectra are shown in Fig. 3a for the resonances of atoms T23Cγ 2 , Q27Cβ and W10Cδ 1 for which 16, 20 and 22 distance correlations are found, respectively. Those correlations are highlighted in the final calculated structure in Fig. 3b along with additional correlations from atoms P6Cδ (12 correlations), P44Cδ (23) and Y60Cα (18). An analysis of the final list of constraints reveals that the distance constraints obtained from the two sparse 13 C-labelling schemes are highly complementary, with <5% of constraints being shared between the 1-Glc and 2-Glc data sets ( Fig. 4b ). Although few cross-peaks are shared between the same atom pairs in the two data sets, the amino-acid pairs giving rise to long-range correlations are highly similar ( Fig. 4d ), providing an independent confirmation that the resonance assignments and preliminary fold are accurate ( Fig. 4a,c ). 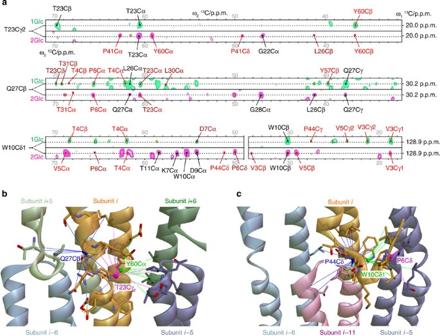Figure 3: Identification of ssNMR contacts leading to high-resolution structural features. (a) PDSD spectra recorded using [1-13C]-glucose-labelled (green) and [2-13C]-glucose-labelled (magenta) MxiH needle samples. Strips are extracted for three indicated resonance positions, corresponding to the assignments of13C nuclei T23Cγ2, Q27Cβ and W10Cδ1. Assigned cross-peak labels are coloured black for intra-residue, dark red for medium-range and light red for long-range atom pair contacts. Ambiguous cross-peaks are marked with a yellow rhombus. (b,c) Converged structural features of the T3SS needle highlighting the quality of ssNMR constraints used, for atoms inb: Q27Cβ from subuniti(blue), T23Cγ2from subuniti(pink) and Y60Cα from subuniti(green), and inc: P44Cδ from subuniti–11(blue), W10Cδ1from subuniti(green) and P6Cδ from subuniti(pink). Figure 3: Identification of ssNMR contacts leading to high-resolution structural features. ( a ) PDSD spectra recorded using [1- 13 C]-glucose-labelled (green) and [2- 13 C]-glucose-labelled (magenta) MxiH needle samples. Strips are extracted for three indicated resonance positions, corresponding to the assignments of 13 C nuclei T23Cγ 2 , Q27Cβ and W10Cδ 1 . Assigned cross-peak labels are coloured black for intra-residue, dark red for medium-range and light red for long-range atom pair contacts. Ambiguous cross-peaks are marked with a yellow rhombus. ( b , c ) Converged structural features of the T3SS needle highlighting the quality of ssNMR constraints used, for atoms in b : Q27Cβ from subunit i (blue), T23Cγ 2 from subunit i (pink) and Y60Cα from subunit i (green), and in c : P44Cδ from subunit i–11 (blue), W10Cδ 1 from subunit i (green) and P6Cδ from subunit i (pink). 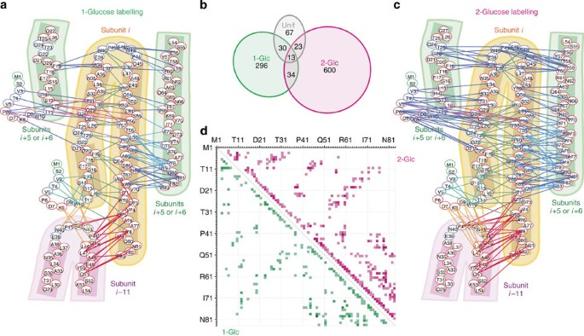Figure 4: Long-range ssNMR constraints detected using two complementary isotopic labelling schemes. Chemical-shift unambiguous long-range constraints identified in (a) [1-13C]-glucose- and (c) [2-13C]-glucose-labelled samples. Inaandcinteractions are colour-coded according to the connecting subunits as follows: green and cyan: intra-subunit; blue, light blue and magenta: interfacei,i±5 ori,i±6; orange and red: interfacei, i±11. (b) Partition diagram of the ssNMR constraints identified in this study considering the different13C-labelling schemes. (d) Residue–residue contact map of the ssNMR constraints, showing medium- to long-range correlations (|i−j|>2) present in the data. Full size image Figure 4: Long-range ssNMR constraints detected using two complementary isotopic labelling schemes. Chemical-shift unambiguous long-range constraints identified in ( a ) [1- 13 C]-glucose- and ( c ) [2- 13 C]-glucose-labelled samples. In a and c interactions are colour-coded according to the connecting subunits as follows: green and cyan: intra-subunit; blue, light blue and magenta: interface i , i ±5 or i , i ±6; orange and red: interface i, i ±11. ( b ) Partition diagram of the ssNMR constraints identified in this study considering the different 13 C-labelling schemes. ( d ) Residue–residue contact map of the ssNMR constraints, showing medium- to long-range correlations ( |i−j|>2 ) present in the data. Full size image Iterative structure calculations using Rosetta We performed a series of Rosetta structure calculations to integrate the ssNMR and cryo-EM data towards determining the final MxiH needle structure. We used an iterative assignment approach that makes use of prior knowledge alongside the structure determination process ( Fig. 2 ). Given the previous analysis of ‘anchor’ constraints ( Fig. 1a ) showing that the preliminary fold and inter-subunit arrangement are similar to the PrgI needle structure [13] for residues L12 to R83, we initialized the assignments of all remaining ambiguous constraints ( Fig. 1b ) using the shortest distance in a homology-based model of MxiH [16] . In the resulting first-round calculations performed using the preliminary ssNMR constraints and cryo-EM density, the lowest-energy models showed convergence to the correct needle fold and subunit arrangement; however, structural convergence in the preliminary ensemble was insufficient to define a high-resolution structure (below 5 Å backbone r.m.s.d.). The 10 lowest-energy models were then used to refine the chemical-shift assignments in the NMR peak lists and the interface assignments of the constraints. We performed two more iterations of structure calculations followed by assignment refinement until structural convergence to below 2.5 Å was reached in the low-energy ensemble. In this process, 194 constraints were discarded from the final constraint data set, as they were found to be inconsistent with a unique interface assignment; either multiple interface assignments were possible or the cross-peaks corresponded to longer than expected distances in the models (as outlined in detail in the Rosetta structure calculations section of Methods). For instance, the increased rigidity of the C-terminal helices [16] can enhance the rate of PDSD. A final refined list of 996 medium- and long-range constraints was obtained from both 1-Glc and 2-Glc data sets, with the following distribution: 580 intra-subunit, 124 inter-subunit, axial and 292 inter-subunit, lateral. Using the refined constraints, we computed 5,000 models ranked according to the weighted sum of Rosetta energy, EM density correlation and ssNMR constraint score terms. The 10 top-ranking models of the final assignment round were converged to below 2.5 Å in backbone r.m.s.d. and showed a minimal number of constraint violations (1.6–3.5%), while also showing good correlation to the EM density (0.62–0.67, see Supplementary Fig. 1 ) and structural statistics according to Rosetta’s energy function. Three models were further selected, each based on different criteria: (1) Rosetta energy, (2) number of constraint violations and (3) correlation to the cryo-EM density. Each of the 3 top-ranking models was further refined 10 times in full-atom mode by optimizing the weights of both the EM density and NMR constraint score terms, as described in the Methods section (see also Supplementary Fig. 2 ). This step was done to evaluate how changes in side-chain packing and local backbone dihedrals (within 1.5 Å backbone r.m.s.d.) affect the energies of different starting models. The final 10 lowest-energy, refined models showed optimal geometry, good fits to the EM density and minimal constraint violations and were deposited in the PDB (PDB ID 2MME and Table 1 ). Table 1 NMR constraint and refinement statistics. Full size table Cross-validation of the structure determination approach Towards an atomic-level validation of the final structure, we employed additional ssNMR data not used at any stage of the iterative calculations and assignment process from two sources ( Table 1 ): 1 H– 1 H correlations from uniformly labelled samples observed in ChhC and NhhC spectra (96 atom-pair correlations) and ambiguous correlations from all three isotopic labelling schemes (595 correlations). The vast majority of these constraints were satisfied in the final ensemble (validation set: 660/691, 4.5±0.1% violations, mean±s.d. over the 10 top-ranking models, protein data bank (PDB ID 2MME), therefore supporting the accuracy of the structure at the atomic level ( Fig. 5a ). Using this unbiased cross-validation approach, we tested whether the previously published structure of MxiH determined using the same cryo-EM data alone [22] (PDB ID 3J0R) was compatible with the experimental ssNMR distance constraints ( Fig. 5b ). Notably, the number of distance violations more than doubles (validation set: 615/682, 9.8% violations). A pairwise comparison of all distances in the validation data set indicates that the models determined using both the ssNMR and cryo-EM data (this study) have significantly shorter distances compared with the previous cryo-EM structure, on average 1.22 Å shorter per distance constraint (paired difference Student’s t -test, 95% confidence level), demonstrating the high accuracy of the hybrid structural determination approach. The median distance for the validation set and pairwise comparison of distances were also used to monitor and guide the modelling procedure between successive rounds of structure calculations, similar to the concept of R free employed in crystallography [31] . 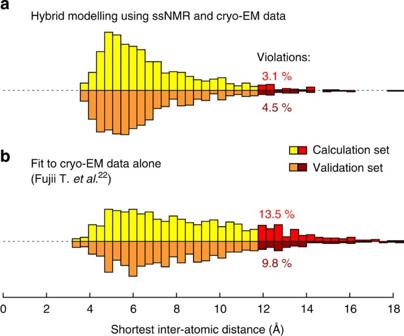Figure 5: Cross-validation of different deposited MxiH needle models. Histogram of shortest identified distances for (a) a final model obtained from the hybrid structure determination approach presented here (PDB ID 2MME) and (b) the model reported by Fujiiet al.22by fitting of the 7.7-Å cryo-EM density map (EMD 5352) alone (PDB ID 3J0R). For each observed cross-peak part of the calculation set (yellow, 996 correlations) and validation set (orange, 691 correlations), the shortest distance is calculated considering all possible chemical-shift assignments within the chemical-shift tolerance window (±0.15 p.p.m. for13C chemical shifts) and all 7 possible subunit assignments (seeFig. 1b). By considering only the shortest distance, this procedure prevents the introduction of any bias in the cross-validation statistics arising from manual peak picking of the ssNMR spectra. The validation set was not used at any time in the structure calculations. Experimentally observed correlations that have an inter-nuclear distance above 12 Å in each model are classified as violations (red histograms). The present model (a) fits the validation data set by an average of 1.22 Å per distance constraint shorter thanb(paired difference Student’st-test, 95% confidence level). Figure 5: Cross-validation of different deposited MxiH needle models. Histogram of shortest identified distances for ( a ) a final model obtained from the hybrid structure determination approach presented here (PDB ID 2MME) and ( b ) the model reported by Fujii et al. [22] by fitting of the 7.7-Å cryo-EM density map (EMD 5352) alone (PDB ID 3J0R). For each observed cross-peak part of the calculation set (yellow, 996 correlations) and validation set (orange, 691 correlations), the shortest distance is calculated considering all possible chemical-shift assignments within the chemical-shift tolerance window (±0.15 p.p.m. for 13 C chemical shifts) and all 7 possible subunit assignments (see Fig. 1b ). By considering only the shortest distance, this procedure prevents the introduction of any bias in the cross-validation statistics arising from manual peak picking of the ssNMR spectra. The validation set was not used at any time in the structure calculations. Experimentally observed correlations that have an inter-nuclear distance above 12 Å in each model are classified as violations (red histograms). The present model ( a ) fits the validation data set by an average of 1.22 Å per distance constraint shorter than b (paired difference Student’s t -test, 95% confidence level). Full size image Verification of sample compatibility and tilt angle In the present application of our hybrid approach, we combine structural constraints obtained from two experimental techniques, where the employed T3SS needle samples also differ in their preparation: for the cryo-EM density map, overexpressed MxiH serotype 2 needles were extracted by shearing from the bacterial surface; for the ssNMR distance constraints, serotype 6 MxiH needles were polymerized in vitro . In the previous sections, we have demonstrated that the hybrid models produced by our approach satisfy the experimental data from both sample preparations: all features of the cryo-EM density map (correlation of 0.62–0.67), including the protrusion region of electron density between subunits ( i ) and ( i −5) (see Supplementary Fig. 1 ), and the independent ssNMR distance constraints. To confirm the compatibility of the samples employed to produce the two data sets, we recommend as part of the hybrid approach the measurement of independent data allowing the validation of the final structure at the macroscopic level. We thus recorded STEM images of in vitro polymerized MxiH needles ( Supplementary Fig. 3 ) to independently identify their helical arrangement. The intensity of scattered electrons in a dark field image is directly related to the mass of the object. We determined the mass-per-length of the polymerized needle assemblies present in the ssNMR samples by integration of needle segments from calibrated STEM images [32] , [33] . Considering the MW of the MxiH subunit protein (9,391 Da MW), the observed mass-per-length of 2,184±2 Da per Å corresponds to an axial subunit displacement of 4.30 Å in the needle assembly. This value is highly consistent with the axial subunit displacement measured in the final hybrid ensemble deposited in the PDB, 4.33±0.02 Å, and confirms that in vitro polymerized needles adopt an 11-start helical symmetry ( Supplementary Fig. 3 ). When viewed from the outside of the structure, the needle filament shows a staggered pattern ( Fig. 6 ), where subunit ( i ) interacts laterally with subunits ( i ±5,6) and axially with subunits ( i ±11). Notably, subunits ( i ) and ( i ±1) are not in close proximity. In the hybrid models ( Fig. 6a ), the subunit ( i +11) does not stack exactly on top of complete of subunit ( i ) as would be predicted for a number of subunits per two turns of precisely N =11.0. Instead, the number of subunits per two turns is N =11.2 and the needle filament accumulates a ‘tilt’ angle of −6.40° (positive in the counter-clockwise direction) for each of the subsequent 11 subunits ( Fig. 6b ). Recently, small changes in the tilt angle of the flagellin proto-filament and in the twist orientation have been shown to be important for the function of the flagellum in bacterial motility [34] . 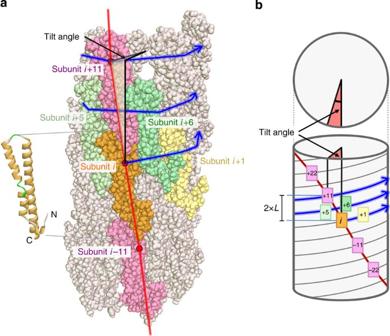Figure 6: Tilt angle of the needle filament. (a) Side view of the hybrid needle structure coloured according to subunit number. The secondary structure of subunit (i) is presented on the left. Blue lines connect successive subunits (i,i+1,i+2,i+3,...) and form a right-handed spiral. The helical axis of the filament is indicated as a bold black line. The red line connects subunits that share an axial interface (i,i+11,i+22,i+33,...). Subuniti+11 (pink) is not directly above subunit (i) as there areN=11.2 protein subunits per two turns of the helix (blue line). As a result, the filament has a slight tilt and the red line forms a slowly rotating left-handed spiral. (b) Schematic representation of the needle filament and tilt angle. The tilt angle (red) is positive in the counter-clockwise direction and can be calculated byα=(360°/N) × (11−N), whereNis the number of subunits per two turns. The axial translation between subunit (i) and subunit (i+11) is indicated (2 ×L). Figure 6: Tilt angle of the needle filament. ( a ) Side view of the hybrid needle structure coloured according to subunit number. The secondary structure of subunit ( i ) is presented on the left. Blue lines connect successive subunits ( i , i +1, i +2, i +3,...) and form a right-handed spiral. The helical axis of the filament is indicated as a bold black line. The red line connects subunits that share an axial interface ( i , i +11, i +22, i +33,...). Subunit i +11 (pink) is not directly above subunit ( i ) as there are N =11.2 protein subunits per two turns of the helix (blue line). As a result, the filament has a slight tilt and the red line forms a slowly rotating left-handed spiral. ( b ) Schematic representation of the needle filament and tilt angle. The tilt angle (red) is positive in the counter-clockwise direction and can be calculated by α =(360°/ N ) × (11− N ), where N is the number of subunits per two turns. The axial translation between subunit ( i ) and subunit ( i +11) is indicated (2 × L ). Full size image Handedness of the helical assembly The new structure determination approach presented here further determines the handedness of the needle super-helix. In the initial PrgI needle calculations [13] , the handedness of the needle could not be defined on the basis of the ssNMR and cryo-EM experimental data alone, as both left- and right-handed geometries gave very similar constraint scores. Subsequent calculations on PrgI needles employing an extended number of ssNMR restraints showed that the needle filament adopts a right-handed geometry [14] . The current ssNMR data for the MxiH needle contains a large set of long-range constraints that should in principle be able to distinguish between the two alternative helical arrangements ( Fig. 7 ). To address this question, the calculations are repeated assuming a left-handed needle, inverting the i +5 and i +6 initial assignments. Notably, the right-handed calculations ( Fig. 7a ) lead to significantly better optimization of the NMR constraints, average of 22.5±1.5 violations per model relative to 37.4±3 for the left-handed calculations ( Fig. 7b ), that can be attributed to fewer violations of lateral constraints. A significant difference is also obtained in the average full-atom energies (−143±15/−93±19 Rosetta energy units in the right- and left-handed low-energy ensembles, respectively), suggesting that the right-handed structures show more favourable side-chain packing and hydrogen-bonding terms. Taken together, these results show that the current hybrid approach can precisely determine the long-range features of the structure, such as its handedness, in addition to the radius, tilt angle and helical pitch parameters consistent with all the available data. 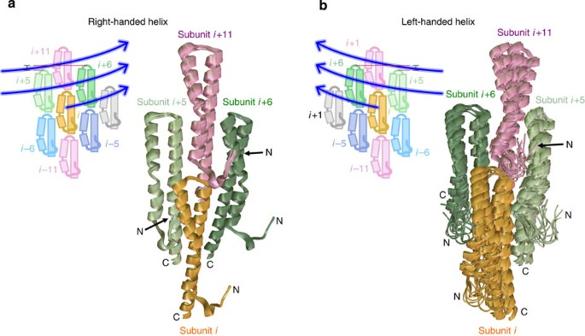Figure 7: Superposition of right-handed and left-handed structural ensembles. The 10 top-ranking models produced by the hybrid structure determination approach considering (a) a right-handed helix and (b) a left-handed helix. The basic tetramer formed by the symmetric subunits (i, orange), (i+5, light green), (i+6, dark green) and (i+11, pink) is presented and the N and C termini are indicated. The relative position of protein subunits is explained schematically in the top-left corner ofaandbfor the two arrangements. In a right-handed helix, the subunit (i+5), closer to (i) in terms of axial translation, is located to the left of (i) while subunit (i+6), further away from (i) is located to the right. Blue lines connect successive subunits as inFig. 6. The right-handed ensemble shows sharper convergence compared with the left-handed ensemble, presents less NMR constraint violations and has a more favourable full-atom Rosetta energy, unequivocally identifying it as the correct handedness. Figure 7: Superposition of right-handed and left-handed structural ensembles. The 10 top-ranking models produced by the hybrid structure determination approach considering ( a ) a right-handed helix and ( b ) a left-handed helix. The basic tetramer formed by the symmetric subunits ( i , orange), ( i +5, light green), ( i +6, dark green) and ( i +11, pink) is presented and the N and C termini are indicated. The relative position of protein subunits is explained schematically in the top-left corner of a and b for the two arrangements. In a right-handed helix, the subunit ( i +5), closer to ( i ) in terms of axial translation, is located to the left of ( i ) while subunit ( i +6), further away from ( i ) is located to the right. Blue lines connect successive subunits as in Fig. 6 . The right-handed ensemble shows sharper convergence compared with the left-handed ensemble, presents less NMR constraint violations and has a more favourable full-atom Rosetta energy, unequivocally identifying it as the correct handedness. Full size image Many important biological assemblies are not amenable to conventional atomic structure determination methods. However, precise knowledge of the structure of biological assemblies is at the foundation of a mechanistic understanding of biological processes, such as bacterial infection. Here, we demonstrate that a hybrid approach ( Fig. 2 ) can determine the structures of molecular assemblies at atomic resolution with high accuracy, by integrating two complementary sources of experimental information, ssNMR and cryo-EM. The new approach has several key advantages relative to the current state-of-the-art structure determination protocols based solely on ssNMR [27] , [28] , [29] : 1 The symmetry of the system is modelled explicitly using a generalized framework [35] recently extended to include helical symmetries [13] . This allows for manipulating the internal backbone and side-chain conformation alongside the rigid-body degrees of freedom for more efficient sampling of conformational space by (a) only considering conformations that are consistent with a given symmetry and (b) performing a minimal number of energy and derivative calculations that are propagated among the different symmetric subunits. This allows us to model the long-range order of the needle filament together with the local atomic structure, which is needed for the use of the cryo-EM density as a calculation bias in addition to the NMR data. 2 Our approach for iterative restraint assignment alongside the structure calculation process is similar to previous NMR structure determination protocols [36] , [37] , further enhanced by the use of a physically realistic, all-atom energy function [38] and extended to supramolecular assemblies with complex symmetries. By using the all-atom energy function to model hydrogen-bonding networks and side-chain packing interactions [39] , our approach does not rely as heavily on the experimental constraints, which are used only as a minor calculation bias with minimal weights to prevent over-fitting. This approach also avoids the need for inferring additional hydrogen-bond constraints not directly observed experimentally, as done in previous ssNMR studies of similar systems [27] , [28] , and is more robust to the exact parameterization of constraint upper limits that can depend on both the system and type of experiment and labelling scheme, as shown extensively in previous work [29] . 3 The combination of the complementary cryo-EM and ssNMR data is crucial in obtaining a converged set of models that are further consistent with the Rosetta energy function. In particular, the cryo-EM density map was necessary for sampling the correct needle topology and subunit arrangement in the early stages of the structure calculations, to verify and extend the initial assignments of the NMR distance constraints ( Fig. 2 ). Finally the 7.7 Å density [22] allows for better defining the rigid-body orientation of the subunits, and calculations performed using the ssNMR restraints alone show higher Rosetta energies relative to the hybrid models. Therefore, by taking advantage of a combination of complementary data sets, the new approach is highly suitable for challenging complexes where either technique alone would be insufficient to uniquely define a high-resolution structure. Different biophysical techniques used in a hybrid approach are likely to have different requirements for sample conditions. For example, the cryo-EM data were obtained on samples of needles sheared from Shigella flexneri culture overexpressing MxiH [22] while the ssNMR data used here were recorded on isotopically labelled samples that were prepared by heterologous bacterial expression and polymerized in vitro . This sample preparation method is necessary to obtain sufficient quantities of labelled MxiH needles needed to record high-resolution NMR spectra [18] . Biochemical, immuno-labelling and biophysical characterization of the needle samples done previously in our group has established that the in vitro reconstituted needles indeed reflect the in vivo needles, as outlined in detail in refs 13 , 16 . Finally, the fact that we obtain convergence on a unique set of models showing good fits to both the cryo-EM density ( Supplementary Fig. 1 ) and satisfy independent ssNMR constraints with only a minimal number of violations ( Table 1 ; Fig. 5 ) further suggests the compatibility of the two data sets at the atomic level. The high-resolution MxiH structure determined here is consistent with the needle architecture established previously [13] , [14] , [16] consisting of 5.6 subunits per turn ( N =11.2) of a 23.5-Å-pitch helix. The radius of the needle is 23.5 Å, consistent with previous EM studies [40] . Moreover, the structure of the non-conserved N terminus (M1-T11) is now fully resolved, showing a short α-helical conformation involving residues P6–D9 (PDKD), which occupies a ‘protrusion’ region of the EM density ( Supplementary Fig. 1 ). The same density region was attributed to an intra-subunit β-sheet in a previously published model using the cryo-EM data alone [22] . The conformation of the N terminus is defined by 132 intra-subunit constraints, including a cluster of constraints connecting V3, W10 and L15 ( Fig. 4a,c ). In addition, there are 46 inter-subunit constraints connecting the N-terminal residues V3–W10 of subunit ( i ) to residues D20–L34 at the N-terminal α-helix of subunit ( i −5), and two correlations between subunits ( i ) and ( i −5), V5–Y57 and P6–Y60, indicate that the beginning of the PDKD motif points inside the needle assembly ( Fig. 3b,c ). Finally, a cluster of three constraints connects T11 of subunit ( i ) to E56 located in the C-terminal (inner) α-helix of subunit ( i −6). The MxiH needle structure highlights key, conserved features involved in the translocation mechanism of substrate proteins ( Fig. 8 ). A recent functional and cryo-EM analysis of MxiH needles using designed trapped substrates showed that effector proteins are translocated in an unfolded state directly through the needle pore in a directional manner [41] . Close inspection of the electrostatic potential on the structure itself reveals that, while the needle lumen presents several charged residues to interact with unfolded substrates, these are typically compensated by conserved opposite charges, resulting in an electrostatically balanced surface ( Fig. 8a,b ). An inspection of the sequence conservation pattern on the MxiH needle structure identifies two clusters of highly conserved residues ( Fig. 8c,d ). While the first cluster forms a continuous patch on the interface between interacting subunits and plays a key role in the structural integrity of the complex ( Fig. 8d , top of the structure), a second cluster of residues Lys 69, Lys 72 and Asp 73 forms a circular arrangement that decorates the needle pore ( Fig. 8d , inset). The side chains of these residues participate in a continuous pattern of symmetry-related electrostatic interactions. A previous systematic alanine-scanning mutagenesis study [42] investigated sequence–function relationships in the MxiH needle. This study showed that mutation of each of these three conserved residues to alanine resulted in functionally defective mutants that cannot invade or lyse host cells, although they still show assembly of relatively intact needle structures that are secretion competent. While K69A and K72A resulted in altered secretion profiles of different substrates, the D73A mutant showed a ‘constitutively on’ phenotype and secreted effector proteins in a deregulated manner without sensing an inducing cell-contact signal. These results are in agreement with the luminal localization of K69 and K72 allowing direct side-chain interactions with the secreted proteins, and further suggest a role of D73 in regulating substrate release from the needle. The availability of the high-resolution MxiH structure produced by the new hybrid methodology now permits the rational design of experiments towards elucidating the mechanism of translocation through the needle pore and the study of interactions between the needle and other components of the T3SS or molecules of the extracellular milieu. 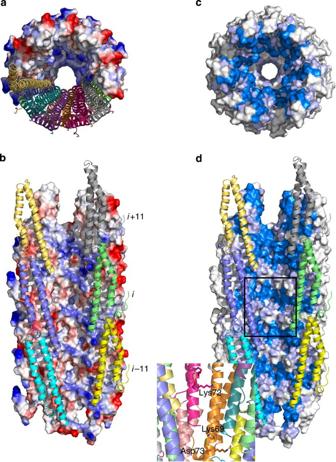Figure 8: Conserved charged residues decorate the MxiH needle pore. (a) Top and (b) side view of the hybrid needle structure showing the surface electrostatic potential computed using APBS58and contoured linearly in the range ±5 kT/e. The helical arrangement of subunits is shown as cartoons for one half of the full 29-subunit system as a guide. Inbandd, three 11-start protofilaments have been removed for simplicity. (c,d) Same view as inaandb, with surface colouring according to the sequence conservation index calculated from the alignment of 102 unique needle sequences using Jalview59, measured on a 1–10 scale. Marine colour indicates high (7–10), light purple medium (4–6) and white low (1–3) sequence conservation index. The boxed region indis enlarged in the inset, indicating the pattern of highly conserved charged residues on the helical structure, as discussed in the main text. Figure 8: Conserved charged residues decorate the MxiH needle pore. ( a ) Top and ( b ) side view of the hybrid needle structure showing the surface electrostatic potential computed using APBS [58] and contoured linearly in the range ±5 kT/e. The helical arrangement of subunits is shown as cartoons for one half of the full 29-subunit system as a guide. In b and d , three 11-start protofilaments have been removed for simplicity. ( c , d ) Same view as in a and b , with surface colouring according to the sequence conservation index calculated from the alignment of 102 unique needle sequences using Jalview [59] , measured on a 1–10 scale. Marine colour indicates high (7–10), light purple medium (4–6) and white low (1–3) sequence conservation index. The boxed region in d is enlarged in the inset, indicating the pattern of highly conserved charged residues on the helical structure, as discussed in the main text. Full size image Sample preparation Three samples of isotopic labelled Shigella flexneri T3SS needles were prepared following the established protocol [13] , [16] for expression, purification and in vitro polymerization of T3SS needle proteins: E. coli strain BL21(DE3) bacteria are transformed with a modified pET16b plasmid containing the mxiH gene fused at the N terminus to a His 7 tag followed by a tobacco etch virus (TEV) protease cleavage recognition sequence. The fusion protein is expressed in minimal medium supplemented with 15 NH 4 Cl as nitrogen source and either [U- 13 C 6 ]-glucose (uniform labelling), [1- 13 C]-glucose (1-Glc labelling) or [2- 13 C]-glucose (2-Glc labelling) as carbon source. The cells are pelleted and lysed. The fusion protein is purified from the lysate by affinity chromatography followed by reverse-phase chromatography. The N-terminal His tag and TEV-cleavage sequence are released after digestion by TEV protease. The MxiH subunit protein is purified by reverse-phase chromatography. The polymerization of MxiH needles was carried out at 37 °C during the 16 days and produced ~20 mg of labelled material each time. Pellets of MxiH needles were obtained by ultracentrifugation at 57,000 g (40,000 r.p.m. at 15 °C during 30 min in a Beckman TL-100.1 rotor), washed 5 × by re-suspending the pellets in fresh buffer and ultracentrifugation and then transferred into 4.0-mm MAS rotors. ssNMR ssNMR experiments were conducted on spectrometers operating at 600 MHz, 800 MHz and 850 MHz 1 H Larmor frequency (Avance I and Avance III, Bruker Biospin, Germany) at MAS rates in the range 10.5–12.5 kHz. The sample temperature was maintained at 5.5 °C by monitoring the temperature using the 1 H chemical shift of water in reference to the methyl 1 H signal of 2,2-dimethylsilapentane-5-sulfonic acid (DSS) [43] . A ramped cross-polarization with contact time of 0.7–1.2 ms was used for the initial 1 H– 13 C and 1 H– 15 N transfers. For 13 C– 13 C correlation experiments, carbon–carbon mixing was accomplished via PDSD with the mixing times ranging from 300 to 850 ms. Experiments with short mixing times (50 or 100 ms) were also recorded to identify intra-residual and sequential correlations. Proton decoupling with a nutation frequency of 83.3 kHz was employed during evolution periods and acquisition, using either SPINAL-64 (ref. 44 ) or SWf-TPPM [45] with a RR supercycle [46] and a tangential sweep [47] ( N =11, sweep window d =0.25, cutoff angle tco=55°, phase angle θ =15°). For spectra recorded on 800 and 850 MHz spectrometers, carbon–nitrogen scalar J couplings were removed by applying c.a. 2 kHz of waltz-16 (ref. 48 ) decoupling on 15 N during acquisition and 13 C evolution periods. On the 600-MHz 1 H frequency spectrometer, spectra were recorded in double-resonance mode to increase sensitivity. Processing and peak picking of ssNMR spectra Spectra were processed using Bruker Topspin 2.1 and the NMRpipe software [49] . A quadratic sine window function is employed in both dimensions, with sine bell shift parameters in the range 3.4–3.8, and Free-Induction-Decay (FID) signals are zero-filled up to the second-next power of two. Polynomial baseline correction was applied in both frequency domains. Spectra were analysed with Sparky [50] (UCSF) and CcpNmr analysis [51] , [52] . We carried out peak picking manually on the basis of our previously reported sequential chemical-shift assignment of MxiH needles [16] (BMRB entry 18651). We first discarded peaks corresponding to artifacts such as spinning sidebands and reflections of the auto-peak diagonal, and we assigned peaks corresponding to intra-residual and sequential correlations, for which cross-peaks are generally also present in short mixing-time PDSD spectra (50–100 ms). Other cross-peaks correspond to medium-range correlations (between residues j and k , 2<| j – k |≤4) or long-range correlations (| j – k |≥5, either intra-molecular or inter-molecular). The average resonance frequency for a given nucleus was obtained from intra-residue and sequential cross-peaks for all spectra or for a single spectral dimension if a sufficient number of cross-peaks are available in one spectrum (>5). To be retained for analysis, a cross-peak must have a signal-to-noise ratio >4.2. The noise in each spectrum is estimated by taking the average of the central 16 out of 20 trials, each trial computing the noise as median of 128 randomly sampled absolute data heights from the spectrum. The median 13 C– 13 C distance detected in PDSD spectra is 6.10 Å, and the 10th- and 90th-percentile distances are 4.37 and 10.08 Å, respectively, a range of distances that is expected for long mixing periods in PDSD spectra ( Fig. 5a ). The constraints detected in ChhC and NhhC spectra involve 1 H– 1 H inter-nuclear distances and therefore offer a higher resolution than the 13 C– 13 C distances obtained from 1-Glc and 2-Glc data sets used in the structure determination process, with a median 1 H– 1 H distance of 5.39 Å, and 10th- and 90th-percentile distances of 4.02 and 8.35 Å, respectively. Assignment of chemical-shift ambiguities For each cross-peak, all resonance assignment possibilities within a tolerance window (0.15 p.p.m. radius of the peak centre for 1-Glc and 2-Glc, 0.2 p.p.m. for uniform labelling) are considered. If only a single possibility exists, the cross-peak is classified as frequency unambiguous. The classification of remaining cross-peaks is done as follows: The method employed here to determine the interface assignment of long-range correlations (either intra-molecular, lateral or axial interface) exploits the different axial translation of subunits ( i ), ( i ±5/6) and ( i ±11), which have 0, ±1 and ±2 axial translation indices with respect to subunit ( i ), respectively ( Fig. 1 ). In particular, for a given cross-peak, assignment possibilities highly incompatible with the preliminary map established based on the symmetric arrangement of the system ( Fig. 1b ) are eliminated. Assignment possibilities incompatible with the isotopic labelling pattern (1-Glc- and 2-Glc-labelled samples) are eliminated as well. For the latter purpose, the basic labelling pattern of glucose-labelled samples was considered [53] , [54] , as well as the additional possibility of scrambling due to subsequent rounds in the citric acid cycle or involvement of other metabolic pathways [20] . The precise labelling patterns for 1-Glc and 2-Glc are confirmed by inference from intra-residual and sequential cross-peaks. If a single assignment possibility remains, the cross-peak is classified as network unambiguous. In the case of multiple remaining possibilities, the cross-peak is classified as network unambiguous only if the average chemical-shift deviation of one assignment is significantly smaller than for other possibilities (at least 0.05 p.p.m. less); otherwise the cross-peak is classified as ambiguous ( Fig. 2 ). Cross-validation procedure The validation set is constituted of cross-peaks not employed at any point of the calculation: ambiguous cross-peaks from 1-Glc and 2-Glc spectra and ambiguous and unambiguous cross-peaks from ChhC and NhhC spectra. Only cross-peaks with a signal-to-noise ratio >6 and corresponding to medium- or long-range correlations were considered. To prevent introducing any bias in the analysis due to the prior constraint assignments, we systematically selected the chemical-shift assignment and the subunit interface giving rise to the shortest inter-nuclear distance within all assignment possibilities contained in the chemical-shift tolerance window. This automatic procedure allows quantifying the agreement of a candidate structure to the experimental ssNMR distance constraints in a completely unbiased and operator-free fashion. An in-house MATLAB program was used to compile the list of shortest distances for an arbitrary PDB file of the needle assembly, yielding the distance distribution histogram ( Fig. 5 ) and median distance. Rosetta structure calculations The structure calculations were performed using the Rosetta symmetric modelling framework [35] extended to helical symmetry [13] . Starting from a helical array of 29 polypeptide chains (83 residues each), the fold-and-dock protocol [55] uses symmetric backbone fragment and side-chain Monte-Carlo trials in internal coordinate space to explore different subunit conformations, and rigid-body moves to explore subunit arrangement that are propagated to symmetry-related subunits according to a user-defined set of transformations. While the MxiH needle ssNMR chemical shifts [16] were used to select 3- and 9-residue backbone fragments [56] , the NMR distance constraints were used to restrain the internal degrees of freedom (backbone dihedral angles and side-chain torsions) together with the 6 rigid-body degrees of freedom that define the relative subunit orientation and helical parameters of the needle filament. We made use of an iterative, structure calculation-guided approach to assign constraints into intra-subunit, and six types of inter-subunit interactions from uniformly labelled samples ( Fig. 2 ). In each round of structure calculations, we used two criteria to assign the raw NMR data interacting atom pairs into the different interfaces and exclude outliers that are consistently violated in the low-energy models: a A constraint was included in the next round if it was satisfied in >30% of the previous round 10 lowest-energy models, according to an absolute upper limit of 12 Å and b a constraint was included in the next round if it can be consistently assigned to the same interface in >70% of the previous round 10 lowest-energy models. While the initial assignments of restraints to the axial ( i to i ±11) and lateral ( i to i ±5 or i ±6) interfaces were based on the secondary structure and symmetry considerations alone, as outlined in the Results section, to initialize the assignments of the lateral interface type, ( i to i ±5 versus i ±6) we made use of limited information from our previously published homology model of the MxiH needle [16] . The structural convergence on a self-consistent network of restraints suggests that our assignment approach leads to the identification of the correct interfaces present in the biological assembly, further confirmed by independent cross-validation ( Table 1 ). This result can be contrasted to the poor assignment and cross-validation statistics obtained using an alternative model [22] (PDB ID 3J0R) of the MxiH needle ( Fig. 5b ). In the more general case, the method can handle completely de novo assignments through the available Rosetta software, as outlined in detail in Supplementary Methods . This circumvents the need for expensive labelling schemes using uniform, diluted and mixed samples described in refs 29 , 30 , and further allows the inclusion of prior knowledge from homologous structures in the PDB, when available. An energy term that measures correlation of the entire 29-subunit system to the 7.7-Å cryo-EM density map was used as described previously [57] to restrain the helical parameters of the needle filament. The EM density and NMR constraint weights were optimized using a grid search in a series of calculations performed with increasing weights while monitoring the total number of violations, EM density fit and Rosetta full-atom energy in the resulting models ( Supplementary Fig. 2 ). NMR constraints were implemented as a flat-bottom potential with an exponential penalty function. The exact values of the 12/9 Å upper limits used in the assignments and final structure calculations, respectively, were calibrated for optimal performance of the method, without using prior structural information. In particular, the 12 Å upper limit was optimal in clearly demarcating wrong assignments from correctly assigned restraints in the early stages of the assignment process, based on a grid search in the range (5–15 Å). The 9-Å limit was based on the observed distribution of 13 C– 13 C cross-peaks in the PDSD spectra relative to the average distances sampled in preliminary structure calculations performed using a 5-Å upper limit. STEM Measurements were carried out at the STEM facility of the Brookhaven National Laboratory (BNL) (Upton, NY, USA). The BNL microscope operates at a voltage of 40 keV and produces a finely focused electron beam of ~0.25 nm in diameter. Three sample preparations were investigated: straight MxiH needles, 3 × diluted needles and 10 × diluted needles, with most images obtained from the 10 × dilution. Tobacco mosaic virus (TMV) particles were added for internal calibration and as a quality control for the sample preparation ( Supplementary Fig. 3 ). The analysis of the images was done using the PCmass 3.2 software (BNL). The default quality-of-fit parameters specified in the software (for example, r.m.s.d. of background pixels, and r.m.s.d. image minus best-fit model) were used to determine the validity of each individual image segment. Image segments are selected for well-separated individual needles in areas of uniform background. The TMV particle segments are fitted with the ‘TMV Rod’ model and the MxiH needle segments are fitted with the ‘9-nm Rod-GC’ model (solid rod). For each scan size (0.512 or 1.024 μm), the size of the integration radius was calibrated for the two fitting models. Accession codes: The final ensemble consisting of the 10 top-ranking models according to Rosetta energy was submitted in the PDB (PDB ID 2MME ). How to cite this article: Demers, J.-P. et al. High-resolution structure of the Shigella type-III secretion needle by solid-state NMR and cryo-electron microscopy. Nat. Commun. 5:4976 doi: 10.1038/ncomms5976 (2014).